Intermolecular [3+3] ring expansion of aziridines to dehydropiperi-dines through the intermediacy of aziridinium ylides The importance of N- heterocycles in drugs has stimulated diverse methods for their efficient syntheses. Methods that introduce significant stereochemical complexity are attractive for identifying new bioactive amine chemical space. Here, we report a [3 + 3] ring expansion of bicyclic aziridines and rhodium-bound vinyl carbenes to form complex dehydropiperidines in a highly stereocontrolled rearrangement. Mechanistic studies and DFT computations indicate that the reaction proceeds through formation of a vinyl aziridinium ylide; this reactive intermediate undergoes a pseudo-[1,4]-sigmatropic rearrangement to directly furnish heterocyclic products with net retention at the new C-C bond. In combination with asymmetric silver-catalyzed aziridination, enantioenriched scaffolds with up to three contiguous stereocenters are rapidly delivered. The mild reaction conditions, functional group tolerance, and high stereospecificity of this method are well-suited for appending piperidine motifs to natural product and complex molecules. Ultimately, our work establishes the value of underutilized aziridinium ylides as key intermediates for converting small, strained rings to larger N- heterocycles. The importance of nitrogenated heterocycles in pharmaceuticals, natural products, and fine chemicals continues to drive innovative strategies for their efficient syntheses from readily available precursors [1] , [2] , [3] , [4] , [5] , [6] , [7] , [8] , [9] , [10] , [11] , [12] , [13] , [14] . The ability to improve upon existing preparations of known compounds, enable alternate retrosynthetic approaches to useful building blocks, and increase opportunities to explore novel chemical space outside of ‘flatland’ are all compelling reasons to develop new approaches to N -heterocycles [15] , [16] , [17] , [18] , [19] , [20] . Piperidines rank as the most prominent N -heterocyclic pharmacophore in current drugs on the market, appearing in ~55% of all FDA-approved drugs containing at least one N- heterocycle, as well as in numerous bioactive natural products [3] . Convergent methods that unite multiple reactive fragments, particularly hetero-[4+2] cycloadditions, deliver substituted dehydropiperidines in enantioenriched form [21] , [22] , [23] , [24] , [25] , [26] , [27] , [28] , [29] , [30] , [31] ; however, critical substrate and/or catalyst control over regio- and stereoselectivity is challenging and often results in narrow scope. Traditional preparations of stereodefined piperidines using intramolecular S N 2-type reactions require selective installation of functional groups prior to ring closure, resulting in lower efficiency, modularity, and step economy as the desired target’s complexity increases [3] . A less common approach is to engage an aziridine and a simple coupling partner in a stereocontrolled, and ideally stereospecific, ring expansion reaction. Aziridines are an ideal starting material for conversion into larger nitrogenated heterocycles. They are easily accessible from a variety of alkenes by nitrene transfer or from simple manipulations of epoxides. In addition, methods for asymmetric aziridination enable these strained rings to be prepared with substantial stereochemical and substitutional complexity [32] , [33] , [34] , [35] , [36] . An attractive feature of aziridines is their ~26 kcal mol −1 of ring strain, ensuring a favorable thermodynamic driving force for ring-opening. 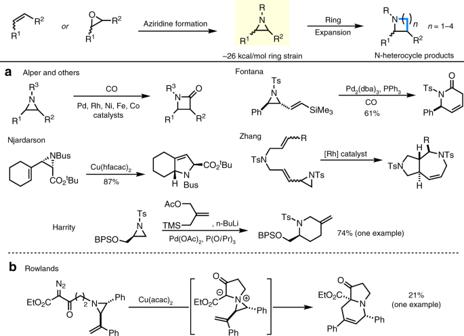Fig. 1: Transformations of aziridines toN-heterocycles. aTypical transition metal-catalyzed ring expansions.bCu-catalyzed aziridine ring expansion through the intermediacy of an aziridinium ylide. Figure 1 illustrates a selection of transition metal-catalyzed aziridine expansions that furnish 4–7 membered N -heterocycles [37] , [38] , [39] , [40] , [41] , [42] , [43] , [44] , [45] , [46] , [47] , [48] . For example, Alper and others have achieved metal-catalyzed carbonylations of aziridines to yield valuable β-lactams, although good regioselectivity depends on the substitution pattern of the three-membered ring [45] . Njardarson has described a series of Cu-catalyzed transformations of aziridines to pyrrolidines and related rings; while these reactions are often stereospecific, they are largely limited to intramolecular examples [40] , [41] , [42] . Scattered examples describing the conversion of aziridines to piperidines, dehydropiperidines, and azepines (Fig. 1a ) are known, but these reactions are also intramolecular or have limited scope [44] , [46] , [47] . In contrast, we were encouraged by Rowlands report of a single example of the formation of a dehydropiperidine in 21% yield (Fig. 1b ) from a vinylaziridine [49] . This reaction presumably occurs through intramolecular formation of an aziridinium ylide, followed by [2,3]-rearrangement; however, only one invertomer undergoes the desired cyclization. The low yield is ascribed to the required coplanarity of the anion and the vinyl group; if the ylide forms with the opposite stereochemistry at nitrogen, [1,5]-hydrogen shifts and other decomposition [50] pathways compete with productive ring expansion. Fig. 1: Transformations of aziridines to N -heterocycles. a Typical transition metal-catalyzed ring expansions. b Cu-catalyzed aziridine ring expansion through the intermediacy of an aziridinium ylide. Full size image As noted in Fig. 1 , aziridines must often be highly engineered to achieve effective ring expansions. In particular, inclusion of an adjacent vinyl group provides the kinetic impetus to drive successful metal-mediated isomerizations and other functionalizations [39] , [40] , [41] , [44] , [46] , [47] . In contrast, utilizing unbiased aziridines for stereocontrolled expansions to larger N -heterocycles can be challenging, as epimerization or racemization of the aziridine must be avoided to successfully relay stereochemical information at sp 3 stereocenters to the product with excellent fidelity [51] , [52] , [53] , [54] . Despite these difficulties, the ease of aziridine preparation and their strain-loaded reactivity make them attractive scaffolds for the discovery of new reactivity [32] , [33] , [34] , [35] , [36] . We previously leveraged the unusual strain (~42 kcal/mol) in methyleneaziridine 1a to achieve a formal [3+1] reaction to furnish methyleneazetidine 1d upon exposure to rhodium-supported carbene 1b (Fig. 2a ) [55] , [56] , [57] , [58] , [59] , [60] , [61] , [62] . Mechanistic studies support initial formation of the aziridinium ylide 1c , which subsequently undergoes a highly asynchronous, concerted [2,3]-Stevens rearrangement to form 1d [63] . The complete transfer of the chirality in 1a – d provides further experimental evidence to support this mechanism. This efficient transformation, which forms new C–C and C–N bonds and two adjacent stereocenters in a stereospecific intermolecular two-fragment coupling, prompted us to undertake further studies of aziridinium ylides to extend the scope to unbiased aziridines. Unfortunately, removing the exocyclic alkene of 1a in 1e (Fig. 2b ) gave only cheletropic extrusion with 1b to furnish 1g , a pathway also observed by Watanabe in Cu-catalyzed reaction of aziridines with ethyldiazoacetate [50] . We reasoned appending a vinyl group to the carbene precursor 1i (Fig. 2c ) could facilitate the desired ring expansion of aziridinium ylide 1j– k over competing cheletropic extrusion to 1l . This transformation represents a net [3+3] annulation of a vinyl carbenoid and a bicyclic aziridine; depending on the mechanism, transfer of stereochemical information from the aziridine to the dehydropiperidine with good fidelity could be envisaged. Herein, we report an attractive strategy to assemble stereochemically complex and highly substituted dehydropiperidines via an intermolecular ring expansion between simple bicyclic aziridines and Rh-supported vinyl carbenes. The intermediacy of an unusual aziridinium ylide species is followed by a stereospecific rearrangement that secures access to enantioenriched products. Fig. 2: Reaction design. a Methyleneazetidines from ring expansion of aziridines. b Competing cheletropic extrusion pathways. c Favoring ring expansion over cheletropic extrusion for the synthesis of dehydropiperidines. Full size image Scope of the [3+3] ring expansion To our delight, reaction of cis -alkene-derived aziridine 2a (Table 1 ) with Davies’ styrenyl diazoacetate [64] 3a under dirhodium catalysis produced 4aa in 75% yield and in excellent >19:1 diastereoselectivity. Optimization of conditions for the [3+3] aziridine ring expansion revealed the dirhodium paddlewheel complex Rh 2 (OAc) 4 was the superior catalyst using slow addition of the vinyl diazoacetate (see the Supplementary Information for further details). With these conditions in hand, the aziridine scope was further explored using 3a as the vinyl carbene precursor. Linear alkyl groups on aziridines 2a–d , including benzyl, methyl, ethyl, and n -butyl, gave good yields of the products 4aa–da in high dr . 1 H NMR spectroscopy indicated a dr of at least >19:1 for the dehydropiperidines, with only trace amounts of the presumed diastereomers noted. Increasing the bulk of the substituent on the aziridine to an isopropyl group in 2e furnished 4ea in 71% yield and excellent dr . Alkyl chloride and ether functionalities were also well tolerated to deliver dehydropiperidines 4fa and 4ga . Alkyl substitution α to the carbamate tether in 2h ( dr > 19:1) gave a 74% yield of 4ha as a single diastereomer. Aziridine 2i , unsubstituted at the terminal carbon, gave 4ia in 67% yield and >19:1 dr . Finally, it was not necessary to have the carbamate contained in a six-membered ring, as the [5.3]-bicyclic aziridine 2j (R 1 = Et, n = 0) gave the [5.6]-bicyclic ring 4ja in 42% yield and in >19:1 dr . Table 1 Scope of the aziridine and diazoester in Rh-catalyzed ring expansions to dehydropiperidines. Full size table We next examined the scope of the carbene precursor using ethyl-substituted aziridine 2c (Table 1 ). The impact of the electronics of a series of phenyl-substituted diazo acetates 3a–f was investigated first. Similar yields were obtained for 4ca and 4cb–cc , irrespective of whether the diazoester carbene precursor contains electron-donating or neutral substituents, highlighting there is little effect of the styrene electronics on the reaction outcome. A single-crystal X-ray structure of 4cc established the relative stereochemical configuration of the heterocycle product (see expansion for 4cc and the Supplementary Information for further details), corroborating nOe studies. Moving the Br to the meta position in 3d resulted in a similar 79% yield of 4cd . Diazoester 3e , bearing a strongly electron-withdrawing trifluoromethyl group, gave a 69% yield of 4ce , also in good dr , providing a convenient way to introduce valuable fluorines into the dehydropiperidine products. Carbene transfer of the naphthyl-substituted 3f provided 4cf in similar yield and dr as compared with 4ca . It was not necessary to employ a styrenyl-derived diazoester, as a series of β-alkyl-substituted diazoesters 3g–i all resulted in good yields of unsaturated piperidines 4cg – ci as single diastereomers as determined by 1 H NMR. The furan-substituted 3j gave 4cj in only 14% isolated yield, as these oxygen heterocycles have been reported to be reactive in the presence of metal-supported carbenoids [65] , [66] . Bulking up the methyl ester on the diazoester to a cyclohexyl ester was also successful, producing 4ck in 56% yield and >19:1 dr . Computational studies of the mechanism The difficulty of studying carbene transfer using traditional kinetics, particularly when slow addition is required, led us to turn to DFT calculations (computational details are in the Supplementary Information and Supplementary Data 1 ) to gain more insight into the mechanism of the ring expansion (Fig. 3 ). The reaction of the methyl-substituted aziridine 2b and the [Rh 2 ]-carbenoid derived from diazoacetate 3a to furnish 4ba was explored computationally. Nucleophilic attack of the aziridine nitrogen atom on the carbon of the Rh-supported carbenoid occurs as the first step to form aziridinium ylide INT1 via transition state TS1 [62] , [63] . Then, barrierless and exergonic dissociation of the dirhodim catalyst from the nitrogen produces zwitterion INT2 , where the negative charge is fully delocalized into the allylic system (Fig. 3b ). Fig. 3: Mechanistic studies of the [3+3] ring expansion. a Computed reaction profile for the process involving 2b and Rh 2 -bound carbene 3a-Rh 2 . Relative free energies (ΔG, computed at 298.15 K and 1 M) and bond distances are in kcal/mol and Å, respectively. All data are computed at the SMD(CH 2 Cl 2 )-B3LYP-D3/def2-SVP level. Values within parentheses are computed at the SMD(CH 2 Cl 2 )-B3LYP-D3/def2-TZVPP//SMD(CH 2 Cl 2 )-B3LYP-D3/def2-SVP level of theory. b Stereochemical retention experiment. Full size image Two fates were envisaged for INT2 . In the first case, INT2 forms azadiene INT3 through a cheletropic extrusion (via TS2 ), followed by a concerted aza-Diels–Alder cycloaddition (via TS3 ) to furnish 4ba . However, subjecting enantioenriched ( S,R ) - 2a [67] to the standard reaction conditions resulted in transfer of the chirality to ( R,R,R )- 4aa with good fidelity (Fig. 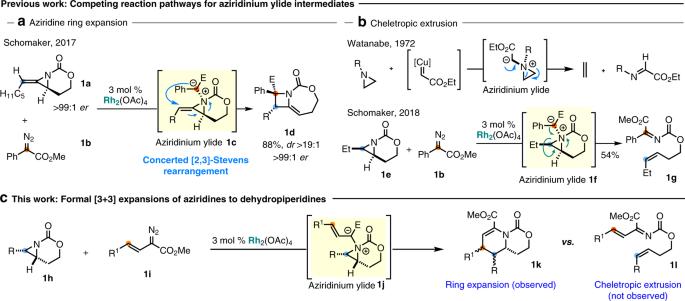Fig. 2: Reaction design. aMethyleneazetidines from ring expansion of aziridines.bCompeting cheletropic extrusion pathways.cFavoring ring expansion over cheletropic extrusion for the synthesis of dehydropiperidines. 3b ). This effectively rules out cheletropic extrusion, followed by aza-Diels–Alder reaction, as the operative mechanism for formation of the dehydropiperidine. We also considered that Stevens rearrangements involving ammonium ylides are occasionally reported to proceed through diradical intermediates [68] ; however, the chirality transfer from ( S,R )- 2a to ( R,R,R )- 4aa suggests that a diradical pathway cannot be operative in the absence of a solvent cage. An alternate fate for the aziridinium ylide INT2 is suggested by the computations in Scheme 3 and involves a rare pseudo-[1,4]-sigmatropic rearrangement of INT2 via TS2′ . This pathway has never been observed for an aziridinium ylide; however, a single example of a [1,4]-rearrangement of an ammonium benzylide has been reported [69] , [70] . According to our calculations, this path proceeds with a lower barrier than the competing cheletropic extrusion (∆∆G ≠ = 5.3 kcal/mol). In addition, this mechanism would be expected to directly parlay absolute and relative stereochemical information from the aziridine into the product, supporting our experimental observations of chirality transfer from ( S,R )- 2a to ( R,R,R )- 4aa [62] , [63] . Zwitterion INT3′ could not be located on the potential energy surface. Indeed, intrinsic reaction calculations (IRCs) starting from TS2′ show the final closing of the C–C bond to form the piperidine exists on a plateau-like energy pathway, where ring closure only begins to occur following completion of the C–N bond rupture. The retention of stereochemistry at the internal aziridine carbon C1 of 2b in 4ba provided an interesting clue to the exact nature of the rearrangement of INT2 to 4ba . One possibility involves intramolecular S N 2 attack of the benzylic carbon on C1 of INT2 (Fig. 3a ) to close the ring. However, it is unlikely a π orbital on the benzylic carbon can overlap effectively with the σ* of the aziridinium ylide to enable S N 2. More importantly, S N 2 attack at C1 would invert the stereochemistry at C1, which is ruled out by the X-ray crystal structure of 4cc . Rather, we propose ring expansion occurs via an unusual stereoretentive nucleophilic substitution; examples of this rare mechanism include the chlorination of secondary alcohols with thionyl chloride (S N i) and benzylic substitution in supramolecular cavities [71] , [72] . Computations also support a stereoretentive ‘S N 1-like’ mechanism. First, the lower energy TS2′ is comprised mainly of C–N bond breakage at the external C1–N bond, which elongates to 1.937 Å. This contrasts to the bond-breaking sequence in the disfavored TS2 , where the internal bicyclic C2–N bond shows more elongation at 2.360 Å, as compared with the C1–N bond (1.735 Å). Thus, even though both TS2 and TS2′ can be described as relatively low-barrier, early transition states, the extent to which the C–N bond breaks appears biased. Second, and consistent with our experimental results, TS2′ predicts that ring opening of the C1–N aziridine bond and the subsequent C–C bond formation must proceed with retention. This is largely due to the stereochemical relationship established between the nitrogen and the carbon substituents of the aziridine during formation of the aziridinium ylide; the carbamate tether controls this stereochemistry and likely plays a key role in restricting the conformational flexibility of the intermediates. Thus, the Me-bearing C1 of the original aziridine 2b is essentially a full carbocation, with nearly complete C–N rupture in TS2′ just prior to stereoretentive ring closure. Chirality transfer The synthetic utility of the sequential nitrene/carbene transfer reaction could be amplified by running it in tandem with asymmetric alkene aziridination to form enantioenriched piperidines over two steps. In 2017, we disclosed an asymmetric aziridination protocol using silver bisoxazoline complexes to enact intramolecular aziridination of homoallylic carbamate esters to achieve high enantioselectivities with a cost-effective catalyst [67] . Application of our asymmetric aziridination to the carbamate of (3Z)-3-penten-5-phenyl-1-ol gave enantioenriched ( S,R ) - 2a [67] in 95:5 er (Figs. 3b and 4a ). Treatment of ( S,R ) - 2a under the standard reaction conditions gives ( R,R,R )- 4aa with minimal loss of ee . Alternatively, a single catalyst could be used to accomplish the sequential nitrene/carbene transfer. Preparation of the allylic N -tosyloxycarbamate ester 5 , according to the method described by Lebel et al. [73] , followed by treatment with Rh 2 (OAc) 4 and K 2 CO 3 generated the intermediate [5.3]-bicyclic aziridine. Filtration and solvent exchange, followed by slow addition of 3a , gave the unsaturated piperidine 4ja in 54% and >19:1 dr . Efforts to identify chemo- and enantioselective Rh-catalyzed aziridination catalysts are underway to secure access to these valuable heterocycles in one pot with good ee . Fig. 4: Tandem nitrene/carbene chemistry and derivatization of products. a Streamlining the nitrene/carbene transfer sequence. b Late-stage functionalization of complex molecules. c Further derivatization of dehydropiperidines. Full size image Functionalization of dehydropiperidine products Further functionalization of the unsaturated piperidine 4ca provides fully substituted, stereochemically rich piperidines in just two steps from the bicyclic aziridine. Indeed, treatment of 4ca with a higher order cuprate furnished 6 in 57% yield and >19:1 dr through a diastereoselective conjugate addition reaction; the relative stereochemistry was verified by both NOE and 1 H NMR-coupling constants (Fig. 4b , see the Supplementary Information for details) [74] , [75] , [76] . In an initial effort to expand the conjugate addition reaction to include other heteroatom nucleophiles, we found treatment of 4ca with DBU and various nucleophiles did not furnish a conjugate addition product, but rather produced styrene 7 in 71% yield and excellent dr (Fig. 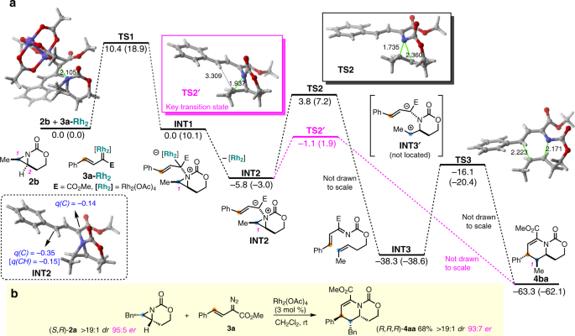Fig. 3: Mechanistic studies of the [3+3] ring expansion. aComputed reaction profile for the process involving2bandRh2-bound carbene3a-Rh2. Relative free energies (ΔG, computed at 298.15 K and 1 M) and bond distances are in kcal/mol and Å, respectively. All data are computed at the SMD(CH2Cl2)-B3LYP-D3/def2-SVP level. Values within parentheses are computed at the SMD(CH2Cl2)-B3LYP-D3/def2-TZVPP//SMD(CH2Cl2)-B3LYP-D3/def2-SVP level of theory.bStereochemical retention experiment. 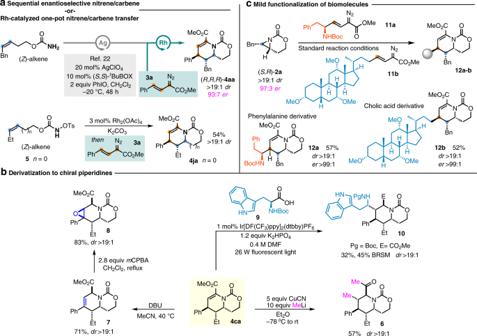Fig. 4: Tandem nitrene/carbene chemistry and derivatization of products. aStreamlining the nitrene/carbene transfer sequence.bLate-stage functionalization of complex molecules.cFurther derivatization of dehydropiperidines. 4b ). Further treatment of 7 with m CPBA yielded epoxide 8 in equally good yield and dr . Furthermore, inspired by MacMillan and coworkers [77] , 4ca was found to undergo a radical Michael addition with Boc-protected tryptophan 9 to yield fully elaborated piperidine 10 in 32% yield as a single diastereomer. Although the yield was modest, this transformation rapidly builds complexity in two steps from a simple aziridine. Finally, the mild reaction conditions and the transfer of the stereochemical information in the aziridine ( S,R )- 2a to ( R,R,R )- 4aa with good fidelity promoted us to explore the potential of this chemistry to append biomolecules to our unsaturated piperidine scaffolds. d -Phenylalanine and cholic acid were transformed into suitable diazoesters 11a and 11b (Fig. 4c ), then subjected to treatment with ( S , R )- 2a (94% ee ) under the standard reaction conditions. The products 12a and 12b were obtained in good yields, with excellent diastereoselectivities and enantiomeric ratios. We envisage this strategy could be effectively applied to explorations of new bioactive chemical space uncovered through fragment-based screening approaches. In conclusion, aziridinium ylides, accessed in high diastereoselectivity from the intermolecular reaction of simple aziridines with metal-bound vinyl carbenes, are shown to be efficient intermediates for the conversion of small ring heterocycles to complex piperidines, a privileged motif in bioactive compounds. DFT computations, in tandem with transfer of chirality experiments, revealed that the ylides undergo a concerted, asynchronous, pseudo-[1,4]-sigmatropic rearrangement to yield products in high diastereoselectivity and with retention of ee installed in the aziridine precursor. Surprisingly, this chemistry bypasses deleterious cheletropic extrusion using unbiased aziridines to give synthetically useful yields of N- heterocycles. In addition, this mechanism proceeds with retention at the C–C bond, a unique consequence of the S N 1-like closing of the vinyl anion tether. We anticipate this report will spur further research into the reactivity of both aziridinium ylides and other onium ylides derived from small-ring heterocycles. General procedure for the dehydropiperidine synthesis A flame-dried round bottom flask is placed under nitrogen and charged with Rh 2 (OAc) 4 (0.03 equiv), followed by a solution of the aziridine (0.1 M in dry CH 2 Cl 2 ). Upon the addition of the aziridine substrate, a color change of green to purple is observed. To this mixture is added a solution of the diazoester compound (1.2 equiv diluted to 0.1 M in CH 2 Cl 2 ) dropwise over 2 h using a syringe pump. The conversion is checked by TLC and 1 H NMR after the addition of the diazoester is complete; once all the starting material is consumed, the reaction mixture is concentrated and loaded directly onto a silica gel column for purification by chromatography using a gradient of 0–50% EtOAc/hexanes.